Rhodobacter capsulatusforms a compact crescent-shaped LH1–RC photocomplex Rhodobacter ( Rba .) capsulatus has been a favored model for studies of all aspects of bacterial photosynthesis. This purple phototroph contains PufX, a polypeptide crucial for dimerization of the light-harvesting 1–reaction center (LH1–RC) complex, but lacks protein-U, a U-shaped polypeptide in the LH1–RC of its close relative Rba. sphaeroides . Here we present a cryo-EM structure of the Rba. capsulatus LH1–RC purified by DEAE chromatography. The crescent-shaped LH1–RC exhibits a compact structure containing only 10 LH1 αβ-subunits. Four αβ-subunits corresponding to those adjacent to protein-U in Rba. sphaeroides were absent. PufX in Rba. capsulatus exhibits a unique conformation in its N-terminus that self-associates with amino acids in its own transmembrane domain and interacts with nearby polypeptides, preventing it from interacting with proteins in other complexes and forming dimeric structures. These features are discussed in relation to the minimal requirements for the formation of LH1–RC monomers and dimers, the spectroscopic behavior of both the LH1 and RC, and the bioenergetics of energy transfer from LH1 to the RC. The genus Rhodobacter ( Rba .) is composed of a highly heterogeneous group of anoxygenic purple nonsulfur phototrophs with 16 validly named species [1] . Among these, Rba . capsulatus along with Rba . sphaeroides have been widely used as models for both fundamental and applied studies in photochemistry, genetics, metabolism, and regulation. Rba . capsulatus in particular has been a workhorse because of its extensive metabolic diversity and facile genetics [2] . According to a recent proposal [1] , [3] , the genus Rhodobacter can be grouped into four major monophyletic clusters based on taxogenomic analyses. Rba . capsulatus falls into Clade II, species of which lack cardiolipin (CL) and glycolipids [1] . By contrast, Rba . sphaeroides falls into Clade I, species of which contain CL and glycolipids and contain larger genomes with higher G + C contents than species in Clade II. The photosynthetic gene cluster in Rhodobacter species contains a unique gene, pufX , which encodes the polypeptide PufX present in the light-harvesting 1–reaction center (LH1–RC) core complex. PufX in Rba . sphaeroides has been demonstrated to play a critical role in dimerization of the LH1–RC complex [4] , [5] , [6] , [7] , [8] , [9] . By contrast, Rba . capsulatus forms only a monomeric LH1–RC despite the presence of PufX [10] , and a similar result has been observed for Rba . veldkampii [11] , [12] , [13] , [14] . In addition, the Rba . sphaeroides LH1–RC contains a newly identified protein named protein-U [8] , [15] (equivalent to protein-Y [7] , [16] or PufY [9] ), while both Rba . capsulatus and Rba . veldkampii lack this protein [15] . The absence of protein-U in a protein-U mutant derivative of Rba . sphaeroides resulted in a reduced amount of the dimeric complex, and the monomeric LH1–RC from this mutant revealed a crescent-shaped structure containing 10–13 αβ-polypeptides (subunits) [8] , [9] ; this compares with the 14 subunits present in the Rba . sphaeroides wild-type monomeric complex [9] , [15] , [16] . Collectively, these data pointed to a crucial role for protein-U in controlling the number of αβ-subunits required for correct assembly and stabilization of the LH1–RC dimer. This conclusion is also supported by a structural analysis of the LH1 from Rba . veldkampii , a protein–U-lacking complex that consists of 15 αβ-subunits and which forms a C-shaped monomeric LH1–RC structure [14] . To further investigate structural and functional roles of protein-U and PufX, we have determined the structure of the native Rba . capsulatus LH1–RC complex. Thus far, no atomic structure is known for either the LH1 or RC from Rba . capsulatus , despite the latter being a well-studied model of purple bacterial photochemistry and spectroscopy [17] , [18] . Surprisingly, and differing from all wild-type LH1s with known structures (obtained from ~10 species), we have found that the current Rba . capsulatus LH1 structure in an RC-associated form contains only 10 αβ-subunits, making it the smallest LH1 complex reported by far. Our results thus reveal that wild-type purple bacteria can produce photosynthetically competent LH1 complexes containing significantly fewer than 14 αβ-subunits and highlights the structural diversity of purple bacterial LH1–RCs. Structural overview The LH1–RC purified from Rba . capsulatus wild-type strain NBRC16435 T using two-step solubilization followed by DEAE chromatography exhibited an absorption maximum ( Q y ) at 882 nm for LH1 (Supplementary Fig. 1 ), and the cryo-EM structure of the core complex was determined at 2.62 Å resolution (Fig. 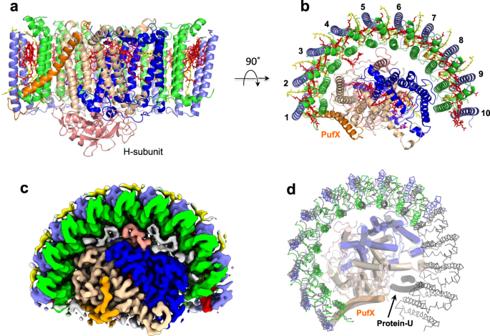Fig. 1: Structure overview of theRba. capsulatusLH1–RC. aSide view of the core complex parallel to the membrane plane. Color scheme: LH1-α, green; LH1-β, slate blue; PufX, orange; RC-L, wheat; RC-M, blue; RC-H, salmon; BChla, red sticks; spheroidenes, yellow sticks; BPhea, magenta sticks.bTop view from periplasmic side of the membrane with the same color scheme as in (a).cTop view of surface representation for the LH1–RC from the periplasmic side. Lipids and detergents are colored in gray.dOverlap view of theRba. capsulatusLH1–RC (colored) and that ofRba. sphaeroides(black, PDB: 7F0L) by superposition of Cα carbons of the RC-M subunits. Protein-U as it exists in theRba. sphaeroidesLH1–RC is shown by a black transparent cartoon. 1 , Supplementary Table 1 and Supplementary Figs. 2 – 5 ). The Rba . capsulatus monomeric LH1–RC forms a crescent-shaped structure with LH1 containing 10 αβ-subunits distributed on one side of the RC with the other side of the RC completely exposed to the membrane region (Fig. 1b, c ). Focused 3-D classification [19] , [20] was conducted iteratively on a localized region containing the gap of the LH1 ring and three αβ-subunits at one end of the LH1 crescent until convergence. Four classes of the 3-D maps were obtained, each of which showed similar conformations independent of resolution (Supplementary Fig. 4 ). By checking these maps, only a single class in each form showed well-resolved density corresponding to the three LH1 subunits, while other maps were relatively featureless yet sufficiently resolved to show that an extra LH1 subunit was not accommodated. Fig. 1: Structure overview of the Rba. capsulatus LH1–RC. a Side view of the core complex parallel to the membrane plane. Color scheme: LH1-α, green; LH1-β, slate blue; PufX, orange; RC-L, wheat; RC-M, blue; RC-H, salmon; BChl a , red sticks; spheroidenes, yellow sticks; BPhe a , magenta sticks. b Top view from periplasmic side of the membrane with the same color scheme as in ( a ). c Top view of surface representation for the LH1–RC from the periplasmic side. Lipids and detergents are colored in gray. d Overlap view of the Rba. capsulatus LH1–RC (colored) and that of Rba. sphaeroides (black, PDB: 7F0L) by superposition of Cα carbons of the RC-M subunits. Protein-U as it exists in the Rba. sphaeroides LH1–RC is shown by a black transparent cartoon. Full size image It is notable that the number of LH1 αβ-subunits is the fewest by far of any core light-harvesting complex from an anoxygenic phototroph. As a result of this small number of LH1 subunits, interactions between LH1 and the RC in Rba . capsulatus are less extensive than those in LH1–RCs composed of a closed or small-gapped LH1 ring where up to 17 LH1 subunits may be present. This was evident from observations that unlike in Rba . sphaeroides , an LH1-only complex was easily isolated from Rba . capsulatus membranes during solubilization and purification (Supplementary Fig. 1a ) and that ~5 % of the isolated complexes were LH1-only (Supplementary Fig. 3a ). PufX is located at one edge of the Rba . capsulatus LH1 crescent and interacts with one pair of αβ-polypeptides and the RC-L subunit (Fig. 1b ). Comparison of the Rba . capsulatus LH1–RC with that of Rba . sphaeroides revealed significant differences. The four LH1 αβ-subunits near protein–U in the Rba . sphaeroides monomeric complex are absent (along with protein-U itself) from the Rba . capsulatus LH1 (Fig. 1d ); this supports the proposed role of protein–U in controlling the number of LH1 αβ-subunits in the Rba . sphaeroides complex [8] , [9] . Many residual densities were observed in the cryo-EM density map of the Rba . capsulatus LH1–RC and assigned to phospholipids and detergents (Supplementary Fig. 6 ). Cofactors in the Rba . capsulatus LH1–RC Twenty-five bacteriochlorophylls (BChl) a , eighteen spheroidenes, two bacteriopheophytins, four ubiquinones (UQ-10) and one nonheme Fe were identified in the Rba . capsulatus LH1–RC (Fig. 2 ). In addition to the BChls a assigned to either LH1 or RC, an isolated BChl a was identified from our cryo-EM density map in the inner space between LH1 and RC on the cytoplasmic side (Fig. 2b ). This BChl a is surrounded by two LH1 α-polypeptides, the RC H-subunit, a phospholipid and a detergent molecule, and is coordinated from the back by a putative myristate at its central Mg (Fig. 2c , Supplementary Fig. 5b ). This “extra” BChl a interacts with nearby Asn52 of the RC H-subunit and Arg15 of an LH1 α-polypeptide through its C13 1 and C13 3 carbonyl groups, respectively, by forming stable hydrogen bonds (Fig. 2c ). Interestingly, the Rba . veldkampii LH1–RC contains an extra bacteriopheophytin (BPhe) a molecule [14] , but its location differs from that of the extra BChl a in the Rba . capsulatus complex (Supplementary Fig. 7 ). Although the function of this extra BChl a in the Rba . capsulatus LH1–RC is unknown, it may play a role in light-harvesting and/or excitation energy transfer considering its nearest distances from an LH1 BChl a (20.8 Å Mg–Mg) and from the accessary BChl a (28.6 Å Mg–Mg) and the BPhe a (21.5 Å edge-to-edge of the macrocycles) in the RC A-branch. Fig. 2: Arrangement of the cofactors in the Rba. capsulatus LH1–RC. a Side view along the membrane plane with the periplasm above and the cytoplasm below. Color scheme: BChl a , red sticks; spheroidenes (group-A), yellow sticks; spheroidenes (group-B), orange sticks; BPhe a , magenta sticks; UQ-10, purple sticks; non-heme Fe, magenta sphere. b Top view from periplasmic side of the membrane with the same color scheme as in ( a ). One additional BChl a and two additional ubiquinones ( Q C and Q D ) were detected in the LH1–RC structure. Arow indicates the extra BChl a . c Close contacts (<4.0 Å) between the extra BChl a and surrounding residues, and Mg–Mg distance between the extra BChl a and the nearest LH1-BChl a . Color scheme as in Fig. 1a except for myristate in gray. d All four of ubiquinones ( Q A , Q B , Q C and Q D ) were detected in the LH1–RC structure. The density maps are shown at a contour level of 5.0 σ . Full size image As for the Rba . sphaeroides LH1 [9] , [15] , [16] , two groups of carotenoids were identified in the Rba . capsulatus LH1 complex (Fig. 2a, b ) and confirmed from their absorption spectra (Supplementary Fig. 1a ). Nine all- trans spheroidenes (group-A) are deeply embedded in the transmembrane region between αβ-subunits while eight all- trans spheroidenes (group-B) protrude on the periplasmic surface. In addition to the conserved UQ-10 at the Q A and Q B sites, two ubiquinones were detected in the Rba . capsulatus LH1–RC structure (Fig. 2b, d ): one ( Q C ) was located close to PufX with its head group pointing to the cytoplasmic side while the second ( Q D ) was present on the membrane-exposed side of the RC with its head group near the periplasmic surface. PufX in the Rba . capsulatus LH1–RC The full-length PufX of Rba . capsulatus contains 78 amino acids (Supplementary Fig. 8 ) in which the N-terminal Met and C-terminal 12 residues were invisible in our cryo-EM density map, presumably due to either post-translational modification or disordered conformation. The expressed Rba . capsulatus PufX is reported to contain 68 residues of molecular mass of 7490 Da [21] , however such was not well resolved in our mass spectroscopic analyses (Supplementary Fig. 8c ). Although the transmembrane domain of Rba . capsulatus PufX shows a helical structure resembling that of PufX from other Rhodobacter species (Fig. 3a ), significantly different conformations were found for the N-terminal region (Fig. 3b ), which is known to play a crucial role in dimerization of the Rba . sphaeroides LH1–RC [6] , [8] , [22] . PufX in the Rba . capsulatus LH1–RC has a “turn-up” conformation in its N-terminal region (Ser2–Asn12) that self-associates with its own transmembrane domain (Trp21–Tyr28) and interacts with nearby LH1 α- and β-polypeptides (Fig. 3c, d ). Sequence comparisons of Rba . capsulatus PufX with that of Rba . sphaeroides , a species that forms both dimeric and monomeric LH1–RCs [7] , [8] , [9] , [15] , [16] , revealed low similarities (Supplementary Fig. 8a ) in the N-terminal region, and this was also true for Rba . veldkampii PufX, which contains a relatively short N-terminus and from which only monomeric LH1–RC has been isolated [12] , [14] . These findings highlight the broad structural diversity of PufX, even within a single genus of purple bacteria, and support the conclusion that the N-terminus of PufX is responsible for forming the dimeric core complex of Rba . sphaeroides [4] , [5] , [6] , [7] , [8] , [9] . Fig. 3: PufX in the Rba. capsulatus LH1–RC. a Superpositions of the Rba. capsulatus PufX (orange) with those from Rba . sphaeroides (cyan, PDB:7VY2) and Rba . veldkampii (gray, PDB: 7DDQ). b Expanded view of the N-terminal regions of PufX marked by the dashed box in ( a ). c Interactions (<4.0 Å) of the PufX N-terminus (orange) with the amino acids in its own transmembrane domain and nearby LH1 α(green)- and β(slate blue)-polypeptides. d Schematic representation of self-association of the PufX N-terminus and interactions with surrounding polypeptides. Full size image The Rba. capsulatus RC As expected from sequence comparisons (Supplementary Fig. 9 ), overall structures of the Rba . capsulatus RC proteins were quite similar to those from Rba . sphaeroides [9] , [15] , [16] , [23] , [24] , with a root-mean-square deviation (RMSD) of 0.42 Å for the mainchain Cα carbons (PDB: 7F0L) (Fig. 4a ). Major cofactors in the Rba . capsulatus RC were generally superimposable with those of the Rba . sphaeroides RC (Fig. 4b ) but exhibited local differences. For example, the distance between the Rba . capsulatus special pair BChls a (P) is 7.65 Å (Mg–Mg distance), shorter than that in Rba . 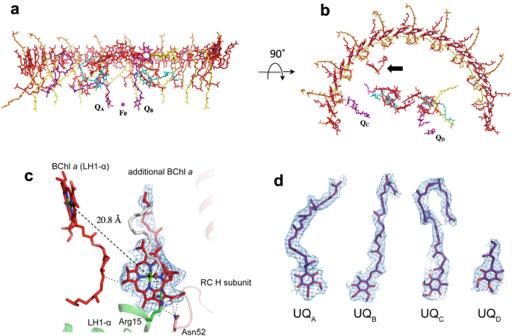Fig. 2: Arrangement of the cofactors in theRba. capsulatusLH1–RC. aSide view along the membrane plane with the periplasm above and the cytoplasm below. Color scheme: BChla, red sticks; spheroidenes (group-A), yellow sticks; spheroidenes (group-B), orange sticks; BPhea, magenta sticks; UQ-10, purple sticks; non-heme Fe, magenta sphere.bTop view from periplasmic side of the membrane with the same color scheme as in (a). One additional BChlaand two additional ubiquinones (QCandQD) were detected in the LH1–RC structure. Arow indicates the extra BChla.cClose contacts (<4.0 Å) between the extra BChlaand surrounding residues, and Mg–Mg distance between the extra BChlaand the nearest LH1-BChla. Color scheme as in Fig.1aexcept for myristate in gray.dAll four of ubiquinones (QA,QB,QCandQD) were detected in the LH1–RC structure. The density maps are shown at a contour level of 5.0σ. sphaeroides (7.85 Å) (Supplementary Table 2 ), whereas the coordination lengths between the ligating His residues and special pair BChls a are longer than those in Rba . sphaeroides (Supplementary Table 2 ). It is also notable that the amino acid adjacent to the special pair BChl a -coordinating His (L174) in the Rba . capsulatus RC-L subunit is a Phe (L173) instead of the Ala present in the Rba . sphaeroides protein (Fig. 4c ). The Phe in Rba . capsulatus lies close (~3.7 Å) to a nearby Trp (L244), enabling π–π interactions between these two aromatic residues (Fig. 4c ). Fig. 4: The RC complex of Rba. capsulatus . a Side view of superposition of Cα carbons for the RC proteins between Rba. capsulatus (colored) and Rba. sphaeroides (gray, PDB: 7F0L). b Cofactor arrangement. Color code: special pair BChl a , red; accessory BChl a , green; BPhe a , cyan; 15- cis -spheroidene, yellow; UQ-10, purple; Fe, magenta. c Structural comparison of the RC-L subunits for the region around the special pair BChl a . Superposition of the Cα carbons of the RC-L subunits between Rba. capsulatus (wheat) and Rba . sphaeroides (gray) shows that the Phe173 (next to the special pair BChl a -coordinating His174) is in close proximity to Trp244. d Structural comparison of the RC-M subunits for the region around the deletion site after conserved Leu105 (arrow head). Superposition of Cα carbons in the RC-M subunits between Rba. capsulatus (blue) and the Rba . sphaeroides ΔU mutant strain (gray, PDB: 7VY3) shows the different arrangement of LH1-α ( Rba. capsulatus , green; Rba . sphaeroides , black ) around the loop between M1 and M2. Viewed from the periplasmic side. Full size image The differences in the special pair BChls a between Rba . capsulatus and Rba . sphaeroides likely contribute to their different absorption maxima. We have measured light-induced P + /P absorption difference spectra of the LH1–RCs purified from Rba. capsulatus and Rba. sphaeroides strain DP2 [25] (Supplementary Fig. 1c ). The absorption maxima of the reduced special pair are at 853 nm for Rba. capsulatus and 871 nm for Rba. sphaeroides in their LH1-assciated forms, indicating that the spectral gap between LH1 and P in Rba. capsulatus (385 cm −1 ) is much larger than that of Rba. sphaeroides (39 cm −1 ). The absorption maxima of the special pairs measured in LH1–RCs are comparable to those measured using the RC-only complexes (~850 nm for Rba . capsulatus [26] and ~865 nm for Rba . sphaeroides [27] , [28] ). The subtle differences in the special pair and surrounding protein environment between Rba . capsulatus and Rba . sphaeroides may also contribute to their different electron transfer rates within the RC. The Rba . capsulatus RC has a faster rate of electron transfer along the B-branch and a slower rate along the A-branch compared with those of Rba . sphaeroides [29] . In this connection, sequence alignment of the RC-M subunits of the two species revealed an insertion (Ala) in the loop between helices M1 and M2 in the Rba . sphaeroides RC-M (Supplementary Fig. 9 ). For this reason, the arrangements of three Rba . capsulatus LH1 α-polypeptides (8th–10th) around this loop deviate from those in Rba . sphaeroides LH1 (Fig. 4d ). Conformational changes in the loop caused by this sequence difference likely induced a different packing arrangement of LH1 and RC in the two species’ core complexes that would be expected to affect electron transfer rates. Due to their close phylogenetic relationship and similar spectroscopic properties, Rba . capsulatus photocomplexes have long been used as alternatives to those of Rba . sphaeroides with the assumption that their corresponding complexes were structurally similar. Although this is generally true for the structurally more conserved RCs, our work has demonstrated that structural differences in the RC-surrounding LH1 complex between these two closely related species are significant and that a broad diversity is possible in the structure of this important component of the photosynthetic apparatus. The crescent-shaped Rba . capsulatus LH1–RC containing 10 αβ-subunits represents a major portion of this complex, and this subunit number is comparable with those of a protein-U-lacking Rba . sphaeroides mutant (strain ΔU) [15] that contains 10–13 αβ-subunits [8] , [9] . The ΔU mutant strain has been demonstrated to grow photosynthetically at a similar rate to that of the wild-type [15] . These findings are supported by kinetic analyses that show that the energy transfer rate from LH1 to the reduced RC in Rba . capsulatus (~2.8 × 10 10 s −1 ) [30] is similar to rates from Rba . sphaeroides (~2.7 × 10 10 s −1 , 14 αβ-subunits) [31] , [32] , Rhodospirillum ( Rsp .) rubrum (1.3–1.7 × 10 10 s −1 , 16 αβ-subunits) [31] , [33] and Thermochromatium ( Tch .) tepidum (1.3–2.0 × 10 10 s −1 , 16 αβ-subunits) [34] , [35] , [36] , [37] . Thus, these data indicate that the energy transfer rate for LH1 → RC (the rate-limiting step in energy trapping from antennae to the RC) is independent of the number of LH1 αβ-subunits ( N ). Similarly, the Rba . capsulatus LH1 structure confirms that the LH1- Q y absorption maximum is also not significantly dependent on the value of N ( Rba . capsulatus Q y = 882 nm versus Rba . sphaeroides Q y = 874 nm and Rsp . rubrum Q y = 877 nm). This agrees with the results of both biochemical analyses and numerical simulation that show that the LH1- Q y for N ≥ 8 were all redshifted to a certain wavelength (around 880 nm at room temperature) with respect to that of monomeric BChl a (~770 nm) [38] , [39] , [40] . Despite extensive efforts, no dimeric LH1–RC has been isolated from Rba . capsulatus (strain Kb-1) [10] or from Rba . veldkampii [12] , [14] , and the same was true in our study using the type strain of Rba . capsulatus (Supplementary Fig. 1c inset). Among multiple factors, PufX has been demonstrated to play a crucial role in dimerization of the Rba . sphaeroides LH1–RC [4] , [5] , [6] , [41] , and its N-terminus has been determined to be directly responsible for the interactions between two monomeric components [6] , [8] , [9] , [22] . The structure in our work here highlights the importance of the PufX N-terminus by showing that the Rba . capsulatus PufX N-terminus adopts a remarkably different conformation from those in other Rhodobacter species with known structures (Fig. 3 ), revealing a significant conformational diversity in this region of the protein. 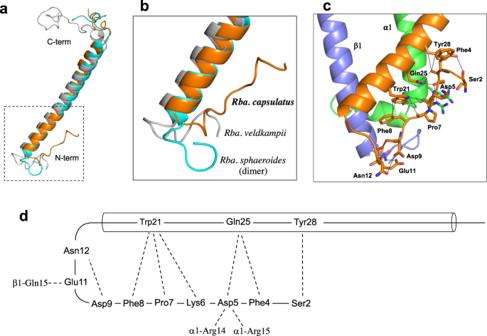Fig. 3: PufX in theRba. capsulatusLH1–RC. aSuperpositions of theRba. capsulatusPufX (orange) with those fromRba.sphaeroides(cyan, PDB:7VY2) andRba.veldkampii(gray, PDB: 7DDQ).bExpanded view of the N-terminal regions of PufX marked by the dashed box in (a).cInteractions (<4.0 Å) of the PufX N-terminus (orange) with the amino acids in its own transmembrane domain and nearby LH1 α(green)- and β(slate blue)-polypeptides.dSchematic representation of self-association of the PufX N-terminus and interactions with surrounding polypeptides. 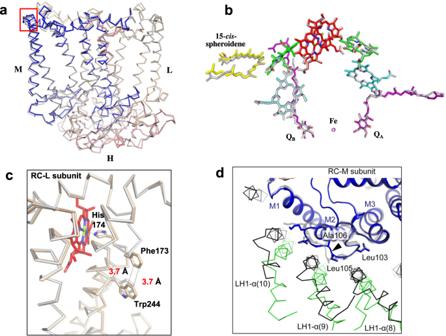Fig. 4: The RC complex ofRba. capsulatus. aSide view of superposition of Cα carbons for the RC proteins betweenRba. capsulatus(colored) andRba. sphaeroides(gray, PDB: 7F0L).bCofactor arrangement. Color code: special pair BChla, red; accessory BChla, green; BPhea, cyan; 15-cis-spheroidene, yellow; UQ-10, purple; Fe, magenta.cStructural comparison of the RC-L subunits for the region around the special pair BChla. Superposition of the Cα carbons of the RC-L subunits betweenRba. capsulatus(wheat) andRba.sphaeroides(gray) shows that the Phe173 (next to the special pair BChla-coordinating His174) is in close proximity to Trp244.dStructural comparison of the RC-M subunits for the region around the deletion site after conserved Leu105 (arrow head). Superposition of Cα carbons in the RC-M subunits betweenRba. capsulatus(blue) and theRba.sphaeroidesΔU mutant strain (gray, PDB: 7VY3) shows the different arrangement of LH1-α (Rba. capsulatus, green;Rba.sphaeroides, black)around the loop between M1 and M2. Viewed from the periplasmic side. This can be understood by the low similarities in overall sequences of PufX (~25% identities for most species) [15] (Supplementary Fig. 8a ) and even lower similarities for their N-termini. Indeed, many of the amino acid residues involved in self-association of Rba . capsulatus PufX (Fig. 3d ) are not conserved [15] . The self-associated conformation of the N-terminus of Rba . capsulatus PufX prevents it from interacting with proteins in another complex, which may explain in part the inability of this species to form a dimeric LH1–RC. Furthermore, the characteristic crescent shape of the 10 αβ-subunit Rba . capsulatus LH1–RC may also inherently weaken its ability to form dimers. This conclusion is supported by our previous work showing that the structure of a monomeric LH1–RC from the Rba . sphaeroides ΔU mutant strain [15] is similar to that of the native LH1–RC from Rba . capsulatus [8] (Supplementary Fig. 10 ) and that the ΔU mutant strain produced a much smaller amount of dimeric LH1–RC than did wild-type cells [15] . Although protein-U in Rba . sphaeroides is unessential for dimerization of LH1–RC, recent studies have shown that protein–U plays an important role in controlling the number of αβ-subunits in an LH1–RC monomer [8] , [9] , [15] , a prerequisite for both LH1–RC dimer formation and stabilization. Rba . capsulatus lacks protein–U, and this likely also contributes to the unique crescent shape of its LH1 and absence of dimeric complexes. The native Rba . capsulatus LH1–RC therefore resembles the monomeric LH1–RC from Rba . sphaeroides mutant strain ΔU in overall structures [8] , [9] (Supplementary Fig. 10 ), with the important distinction that the four αβ-subunits absent from the Rba . capsulatus LH1 are present in Rba . sphaeroides and associate closely with protein-U in its native Rba . sphaeroides LH1–RC (Fig. 1d ). Thus, our Rba . capsulatus LH1–RC structure provides further evidence that interaction of protein–U with up to four surrounding αβ-subunits is a major mechanism for regulating the number of subunits in the Rba . sphaeroides LH1 complexes. This reflects a long-range interaction over a distance of ~ 23 Å (between protein–U and the 11th α-polypeptide) in Rba . sphaeroides . In addition to the effect of protein–U, characteristic interactions between the Rba . capsulatus RC-M subunit and nearby LH1 α-polypeptides may also contribute to the unique crescent shape of its LH1. To better elucidate interaction patterns between the M subunit and nearby LH1 α-polypeptides (8th–10th), we mapped interactions of each LH1 α-polypeptide with different colors onto the surface of the M-subunit (Supplementary Fig. 11 ). In particular, the loop between membrane helices M1 and M2 in the RC-M subunit extensively affects contacts between the M subunit and LH1 α-polypeptides (Supplementary Fig. 11 ). As a result, the reduced arc size of the Rba . capsulatus LH1 weakens its interactions with the RC. This likely explains our ease in isolating an LH1-only complex from photosynthetic membranes of this species during purification (Supplementary Fig. 1 ) and the results of cryo-EM 3-D classification that showed approximately 5% of all particles to consist of LH1-only complexes (Supplementary Fig. 3a ). Although the smallest native LH1 complex yet discovered, the crescent-shaped Rba . capsulatus LH1 structure containing 10 αβ-protein subunits and 37 pigments (20 BChl a and 17 spheroidenes) will still provide a challenging target for the rapidly developing tools of protein structure prediction based on artificial intelligence, as represented by AlphaFold2 (AF2) [42] . This algorithm has offered up many promising results with impressive accuracy for the monomeric and oligomeric protein structures composed of a single polypeptide chain [43] , [44] , [45] . Recent AF-Multimer and other packages derived from AF2 have succeeded in predicting structures of several multimeric protein complexes but are still only applicable to the homo-oligomer or hetero-oligomer consisting of a few protein components [46] , [47] . In order to increase the probability of successfully predicting the structures of hetero-oligomer-containing cofactors, implementation of multimer templates with cofactors and self-distillation approaches is unavoidable, and for such purposes, LH1 structures with variable ring sizes and optimal number of pigments from Rhodobacter species are perfect model systems. When the next generation of prediction tools emerges, it might be possible to deduce the minimal structural requirements for an LH1 complex based on its amino acid sequences and pigment types. Such capability would greatly accelerate progress in dissecting the complex details of the light reactions of photosynthesis—redox biochemistry that ultimately supports all life on Earth. Preparation and characterization of the LH1–RC complex A culture of Rba. capsulatus NBRC16435 (type strain of the species, ATCC 11166 = DSM 1710 = NCIB 8254) was purchased from National Institute of Technology and Evaluation, Japan. Cells were cultivated phototrophically (anoxic/light) at room temperature for 5 days under incandescent light (60 W). Chromatophores (ICM) at OD 850-nm = 40 were treated with 0.25% w/v lauryldimethylamine N -oxide in 20 mM Tris-HCl (pH 7.5) at room temperature for 60 min to remove excess LH2, followed by ultracentrifugation at 150,000× g at 4 °C for 90 min. LH1–RC complexes were solubilized from the pellets by 1.0% n -dodecyl β-D-maltopyranoside (DDM) at room temperature for 60 min in the same buffer, followed by ultracentrifugation at 150,000 × g at 4 °C for 90 min. The crude LH1–RC complexes were loaded onto a DEAE column (Toyopearl 650S, TOSOH) equilibrated at 8 °C with 20 mM Tris-HCl buffer (pH 7.5) containing 0.1% w/v DDM. The fractions were eluted in an order of residual LH2, LH1-only and LH1–RC by a linear gradient of CaCl 2 from 0 mM to 100 mM. The LH1–RC and LH1-only fractions were collected and concentrated for absorption and circular dichroism (CD) measurements (Supplementary Fig. 1 ). LH1–RC complexes were assessed by negative-stain EM using a JEM-1011 instrument (JEOL) (Supplementary Fig. 2a ). CD spectra were recorded on a Jasco J-720w spectropolarimeter in a range of 400–1000 nm under the conditions of 100 nm/min scan speed, 5 nm bandwidth, 1 sec response time and 5 repeated scans [48] . Light-induced P + /P absorption difference spectra of the LH1–RCs were obtained using a V-780 Spectrophotometer (JASCO) by subtracting spectra in the dark from those measured during 940 nm LED illumination at room temperature. Masses of the LH1 polypeptides were determined by matrix-assisted laser desorption/ionization time-of-flight mass spectroscopy (MALDI-TOF/MS) [49] on a 4800 Plus MALDI TOF/TOF Analyzer (Applied Biosystems, MDS SCIEX) equipped with a nitrogen laser (337 nm). Sinapinic acid (3, 5-dimethoxy-4-hydroxy cinnamic acid) was used as matrix and was dissolved in 80% acetonitrile solution containing 0.3% TFA. Typically, the amount of LH1–RC analyzed was of 10–30 pmol. Purified LH1–RC was dissolved in 80% acetonitrile solution containing 0.1% TFA and mixed with the sinapinic acid solution in a ratio of 1:1(v/v) and then loaded onto sample stage for co-crystallization. Analysis was performed in positive and linear modes with typical laser intensity of 4150 and total 1500 shots per spectrum using 4000 Series Explore Software Version 3.5. Phospholipids in intracytoplasmic membranes were analyzed (Supplementary Fig. 6 ) by 31 P-NMR [50] . The extracted phospholipids were dissolved in 500 μL of chloroform- d and mixed with 200 μL of methanol and 50 μL of 0.2 M K-EDTA solution (pH 6.0). 31 P-NMR spectra were recorded at room temperature on a Bruker Biospin Avance III 500 MHz spectrometer equipped with a 5-mm broadband probe tuned to the 31 P nucleus frequency at 202.46 MHz using TopSpin software (ver. 3.6.2). The 31 P-NMR spectra were acquired using inverse-gated proton decoupling (500.13 MHz) with the following parameters: 12,175 Hz sweep width, 30° pulse, 8 K data points, 0.34-s acquisition time, 1.0-s delay time and 2000 scans. 31 P chemical shifts were referred to the peak of 85% H 3 PO 4 . Calibration of the 31 P-NMR signals was carried out using a standard phospholipids kit (Doosan Serdary Research Laboratories, Canada) containing 10 phospholipids. Cryo-EM data collection Proteins for cryo-EM were concentrated to ~3.8 mg/ml. Two and half microliters of the protein solution were applied on a glow-discharged holey carbon grid (200 mesh Quantifoil R2/2 molybdenum), which had been treated with H 2 and O 2 mixtures in a Solarus plasma cleaner (Gatan, Pleasanton, USA) for 30 s and then blotted and plunged into liquid ethane at –182 °C using an EM GP2 plunger (Leica, Microsystems, Vienna, Austria). The applied parameters were a blotting time of 6 s at 80% humidity and 4 °C. Data were collected on a Titan Krios (Thermo Fisher Scientific, Hillsboro, USA) electron microscope at 300 kV equipped with a Falcon 3 camera (Thermo Fisher Scientific) (Supplementary Fig. 2b ). Movies were recorded using EPU software (Thermo Fisher Scientific) at a nominal magnification of 96 k in counting mode and a pixel size of 0.820 Å at the specimen level with a dose rate of 0.846 e-per physical pixel per second, corresponding to 1.26 e-per Å 2 per second at the specimen level. The exposure time was 31.8 s, resulting in an accumulated dose of 40 e-per Å 2 . Each movie includes 40 fractioned frames. Image processing All of the stacked frames were subjected to motion correction with MotionCor2 [51] . Defocus was estimated using CTFFIND4 [52] . All of the picked particles using the crYOLO [53] were further analyzed with RELION 3.1 [54] , and selected by 2-D classification (Supplementary Fig. 2c , and Supplementary Table 1 ). An initial 3-D model was generated in RELION, and the particles were divided into four classes by 3-D classification resulting in only one good class. The 3-D auto refinement without any imposed symmetry (C1) produced a map at 2.67 Å resolution, after contrast transfer function refinement, Bayesian polishing, masking, and post-processing. Then particle projections were further subjected to subtraction of the detergent micelle density followed by 3-D auto refinement to yield the final map with a resolution of 2.62 Å according to the gold-standard Fourier shell correlation (FSC) using a criterion of 0.143 (Supplementary Fig. 3 ) [55] . The local resolution maps were calculated on RESMAP [56] . Focused 3-D classification [19] , [20] was conducted for the gap region of the LH ring as well as three LH1 subunits at the open terminal end in an LH1–RC monomer using the mask [57] in RELION until convergence. Model building and refinement of the LH1–RC complex The atomic model of the Rba . sphaeroides LH1–RC (PDB: 7F0L) was fitted to the cryo-EM map obtained for the Rba . capsulatus LH1–RC using Chimera [58] . Amino acid substitutions and real space refinement for the peptides and cofactors were performed using COOT [59] . Whole regions of PufX and protein–U as well as both terminal regions of the LH1 α-subunit were modeled ab initio based on their density. The manually modified model was refined in real-space on PHENIX [60] , and the COOT/PHENIX refinement was iterated until the refinements converged. Finally, the statistics calculated using MolProbity [61] were checked. Figures were drawn with the Pymol Molecular Graphic System (Schrödinger) [62] , UCSF Chimera [58] , and ChimeraX [63] . Reporting summary Further information on research design is available in the Nature Portfolio Reporting Summary linked to this article.